Hepatitis C virus genetics affects miR-122 requirements and response to miR-122 inhibitors Hepatitis C virus (HCV) replication is dependent on a liver-specific microRNA (miRNA), miR-122. A recent clinical trial reported that transient inhibition of miR-122 reduced viral titres in HCV-infected patients. Here we set out to better understand how miR-122 inhibition influences HCV replication over time. Unexpectedly, we observed the emergence of an HCV variant that is resistant to miR-122 knockdown. Next-generation sequencing revealed that this was due to a single nucleotide change at position 28 (G28A) of the HCV genome, which falls between the two miR-122 seed-binding sites. Naturally occurring HCV isolates encoding G28A are similarly resistant to miR-122 inhibition, indicating that subtle differences in viral sequence, even outside the seed-binding site, greatly influence HCV’s miR-122 concentration requirement. In addition, we found that HCV itself reduces miR-122’s activity in the cell, possibly through binding and sequestering miR-122. Our study provides insight into the interaction between miR-122 and HCV, including viral adaptation to reduced miR-122 bioavailability, and has implications for the development of anti-miR-122-based HCV drugs. The hepatitis C virus (HCV) is a hepatotropic virus that has infected ~3% of the world’s population [1] . Chronic, life-long HCV infection can have severe health consequences, including hepatitis, cirrhosis and hepatocellular carcinoma. The effectiveness of HCV therapies will probably improve dramatically in the next few years with the release of drugs that target both viral and cellular factors. Efficacy against a range of HCV genotypes, side effects and the capacity to elicit viral resistance remain critical issues that necessitate the need for alternative or complementary therapies [2] . The liver-specific microRNA (miRNA) miR-122 is an essential host factor in the HCV lifecycle; however, the mechanism by which miR-122 promotes HCV replication is not fully understood [3] . Although most miRNAs inhibit gene expression by destabilizing the messenger RNA transcripts that they bind, it has been shown that miR-122 binds to two distinct sites in the first 42 nucleotides of the HCV genome, which enhances HCV replication, at least in part by stabilizing the virus’s RNA genome [4] , [5] , [6] , [7] , [8] , [9] , [10] . Treatment with Miravirsen, a locked nucleic acid (LNA) oligonucleotide that binds and antagonizes miR-122, effectively inhibits HCV replication in chimpanzees and humans [11] , [12] . In a phase 2a study, Miravirsen treatment alone resulted in a sustained, dose-dependent HCV decrease in the majority of treated patients, five of whose viral loads fell below detectable levels and one of whose viral loads remained undetectable at the conclusion of the study, 12 weeks after treatment cessation [12] . Although the results from this trial are promising, important questions remain about the use of Miravirsen as a stand-alone therapy or as part of a drug cocktail, including whether drug-resistant viruses will emerge. While this human clinical trial stated that Miravirsen-resistant viruses were not found, a poor understanding of what a resistant virus would look like complicates their detection. Although no mutations were identified in the HCV miR-122-binding sites during or after treatment, it remains possible that sequence changes outside of these sites may impact Miravirsen sensitivity. The fact that not all patients responded to Miravirsen therapy (even at the highest dose, three out of eight patients did not exhibit greater than 50-fold reductions in viral loads), suggests that either host or viral factors influence treatment response. Moreover, the mechanisms by which miR-122 coordinates the HCV life cycle are not completely known, including the quantity of miR-122 required for HCV replication, which further complicates the application of miR-122 antagonists in patient treatment. Here we sought to understand how miR-122 inhibition influences HCV replication over time. We identify a viral variant in which a single nucleotide change in the HCV 5′-untranslated region (UTR), between the miR-122 seed-binding sites, allows the virus to replicate efficiently in the presence of stable miR-122 knockdown. Stoichiometric analysis revealed that although replication of this variant still depends on miR-122, it requires substantially lower levels of miR-122 activity, probably because it can more efficiently bind this miRNA. Furthermore, HCV isolates that naturally encode this sequence also show resistance to miR-122 inhibition, indicating that HCV is sensitive to miR-122 bioavailability in a strain-specific manner. These studies provide quantitative insight into the relationship between miR-122 and HCV, and have implications for the future use of Miravirsen and other miR-122-based drugs for the treatment of HCV infection. Isolating HCV mutant that replicates in miR-122-decoy cells In previous work, we showed that introduction of the miR-122 decoy into Huh-7.5 cells, a hepatocyte cell line that expresses high levels of miR-122, blocked HCV’s ability to replicate in the cells for more than 18 days [13] . To determine how effectively the miR-122 decoy inhibits miR-122 activity, we established Huh-7.5 cell lines expressing a miR-122 sensor ( Supplementary Fig. 1a,b and 3a ). Transduction of increasing doses of decoy led to a de-repression of the sensor that was similar to or greater than the de-repression induced by transfection of a Miravasen like anti-miR-122 LNA, indicating that the miR-122 decoy is at least as effective as LNAs at reducing miR-122 activity ( Supplementary Fig. 1c,d and 3b ). The miR-122 decoy provided an opportunity to examine HCV replication in cells where miR-122 activity is stably reduced. Huh-7.5 cells expressing either a decoy against miR-122, or miR-142 as a negative control (both marked by green fluorescent protein (GFP)), were mixed with naive Huh-7.5 cells, which serve as a susceptible HCV feeder population. The cells were infected with a genotype 2a chimeric HCV (termed Jc1) at a low multiplicity of infection and passaged for several weeks ( Fig. 1a ). Following each passage, the proportion of decoy-expressing and HCV-infected cells was monitored by flow cytometry analysis of decoy-associated GFP and HCV non-structural protein 5A (NS5A) expression. At four days post infection, non-decoy-expressing cells in both populations were efficiently infected with HCV (GFP negative, NS5A positive), demonstrating similar permissivity of these cells ( Fig. 1b ). miR-142 decoy-expressing cells (GFP positive) supported HCV infection as efficiently as the decoy-negative cells at early time points, and HCV infection of this cell population waned over time as HCV non-permissive cells emerged ( Fig. 1b,c ). As expected, miR-122 decoy cells initially did not support efficient viral replication ( Fig. 1b,d ). However, after 26 days, the majority of the miR-122 decoy cells were NS5A positive, suggesting that the virus had gained the ability to replicate in cells in which miR-122 was inhibited ( Fig. 1d ). 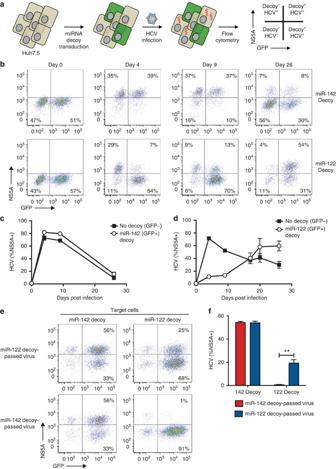Figure 1: Isolation of miR-122-decoy-resistant HCV. (a) Schematic of screen for isolation of mutant HCV. (b) Huh-7.5 cells expressing decoys (GFP positive) for miR-122 or miR-142 (control) were mixed with naive Huh-7.5 cells and infected with WT Jc1. Samples were monitored for the proportion of decoy-expressing and HCV-infected cells by fluorescence-activated cell sorting (FACS) analysis of GFP and HCV NS5A expression, respectively. Quantification of HCV infection in decoy-expressing (open circles) or naive (dark squares) cells in (c) miR-142 decoy or (d) miR-122 decoy-expressing cell populations. (e,f) Infection of fresh miR-122 or miR-142 decoy-expressing cells with virus passaged in miR-122 or miR-142-inhibited cells. FACS plots (b,e) are representative of three independent experiments. Values (c,d,e) represent means and s.d. of triplicate infections. Data were analysed using an unpaired student’st-test, *P<0.05, **P<0.005, ***P<0.0005. Figure 1: Isolation of miR-122-decoy-resistant HCV. ( a ) Schematic of screen for isolation of mutant HCV. ( b ) Huh-7.5 cells expressing decoys (GFP positive) for miR-122 or miR-142 (control) were mixed with naive Huh-7.5 cells and infected with WT Jc1. Samples were monitored for the proportion of decoy-expressing and HCV-infected cells by fluorescence-activated cell sorting (FACS) analysis of GFP and HCV NS5A expression, respectively. Quantification of HCV infection in decoy-expressing (open circles) or naive (dark squares) cells in ( c ) miR-142 decoy or ( d ) miR-122 decoy-expressing cell populations. ( e , f ) Infection of fresh miR-122 or miR-142 decoy-expressing cells with virus passaged in miR-122 or miR-142-inhibited cells. FACS plots ( b , e ) are representative of three independent experiments. Values ( c , d , e ) represent means and s.d. of triplicate infections. Data were analysed using an unpaired student’s t -test, * P <0.05, ** P <0.005, *** P <0.0005. Full size image To determine whether a miR-122 decoy-resistant HCV had emerged, supernatants from miR-122 and miR-142 decoy cultures were passed on to fresh decoy-expressing Huh-7.5 cells. Strikingly, although both passed viruses efficiently infected cells expressing the miR-142 decoy, only the miR-122 decoy-passed virus efficiently infected the miR-122 decoy-expressing cells ( Fig. 1e,f ). These results indicate that the virus passed through miR-122 decoy-expressing cells had gained the capacity to replicate in cells in which miR-122 activity is inhibited. HCV encoding G28A replicates in miR-122-decoyed hepatocytes We sought to understand how the emergent HCV was able to replicate in the miR-122-decoyed cells. We hypothesized that mutations in the HCV genome may have been responsible. To investigate this possibility, we used next-generation sequencing technology to sequence complete viral genomes from viral RNA isolated from the supernatants of three independently passaged viruses ( Fig. 2a ). Variant frequency analysis revealed that the only consistent change was a single G to A mutation at nucleotide 28 of the viral genome (G28A) ( Fig. 2b,c ). Our sequencing achieved 23 × coverage of this position of the genome as well as an average base quality of 35.22±2.04. We confirmed the G28A mutation in the resistant viruses by performing 5′ rapid amplification of complementary DNA ends on the isolated viral RNA. All of the 18 clones sequenced from the 3 independent miR-122 decoy-passed viruses encoded the G28A mutation ( Fig. 2d ). Interestingly, this nucleotide position falls between the two miR-122 seed-binding sites ( Fig. 2e ) and has not been reported to participate in miR-122 binding [4] , [5] , [6] , [9] . Importantly, this change was not found in viruses passaged in miR-142 decoy cells. 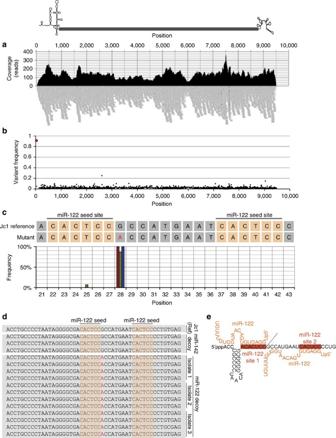Figure 2: Identification of G28A mutation. (a) Illustration of the HCV genome with sequencing read coverage frequency (black contour) and alignment of reads (grey bars), data merged from reads of three isolates. (b) Non-reference variant frequencies identified across HCV genome, red point corresponds to position 28. (c) Mutation position and frequency in each replicate (red bar, isolate 1; green bar, isolate 2; blue bar, isolate 3). (d) 5′-Rapid amplification of cDNA end sequencing of miR-142 decoy- and miR-122 decoy-passed viruses, nucleotides 1-50 of the HCV genome aligned to Jc1 reference. Representative sequences shown. (e) Illustration of Jc1 HCV 5′-UTR (black text) showing the miR-122 binding seed-binding sites (red boxes), miR-122 molecules (orange text) and the position of the G28A mutation that falls between the two miR-122 seed sites. Figure 2: Identification of G28A mutation. ( a ) Illustration of the HCV genome with sequencing read coverage frequency (black contour) and alignment of reads (grey bars), data merged from reads of three isolates. ( b ) Non-reference variant frequencies identified across HCV genome, red point corresponds to position 28. ( c ) Mutation position and frequency in each replicate (red bar, isolate 1; green bar, isolate 2; blue bar, isolate 3). ( d ) 5′-Rapid amplification of cDNA end sequencing of miR-142 decoy- and miR-122 decoy-passed viruses, nucleotides 1-50 of the HCV genome aligned to Jc1 reference. Representative sequences shown. ( e ) Illustration of Jc1 HCV 5′-UTR (black text) showing the miR-122 binding seed-binding sites (red boxes), miR-122 molecules (orange text) and the position of the G28A mutation that falls between the two miR-122 seed sites. Full size image To confirm that the G28A transition was responsible for conferring viral resistance to miR-122 inhibition, we engineered the G28A change in the parent Jc1 genome and tested its ability to replicate in miRNA decoy-expressing Huh-7.5 cells. As expected, wild-type (WT) Jc1 efficiently infected naive Huh-7.5 cells, but was unable to efficiently replicate in miR-122 decoy-expressing (GFP positive) cells, which confirmed that miR-122 was effectively inhibited in these cells ( Fig. 3a ). The G28A mutant was able to replicate as efficiently as the WT Jc1 in naive Huh-7.5 cells, indicating that this mutation does not affect HCV replication in the presence of normal miR-122 levels. Strikingly, the G28A mutant virus also replicated in Huh-7.5 cells expressing the miR-122 decoy ( Fig. 3a ), demonstrating that a single mutation in the HCV genome enhanced replication in the setting of miR-122 decoy expression. To our knowledge, this is the first evidence that an HCV variant can replicate under these conditions, and may be a means for Jc1 to adapt to combat anti-miR-122 therapy. 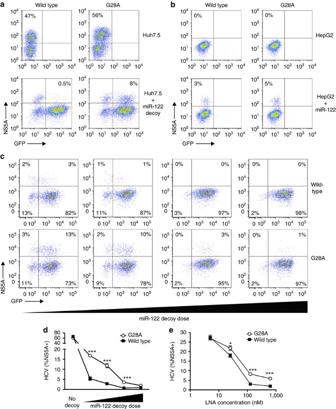Figure 3: G28A mutation renders Jc1 more resistant to miR-122 inhibition than WT. Analysis of HCV (NS5A) infection by fluorescence-activated cell sorting in (a) miR-122 decoy-expressing or naive Huh-7.5 cells transfected with WT or G28A mutant Jc1 RNA, (b) naive or miR-122-expressing HepG2 cells transfected with WT or G28A mutant Jc1 RNA and (c) Huh-7.5 cells expressing increasing amounts of miR-122 decoy infected with WT (top panels) or G28A mutant (bottom panels) Jc1. (d) Quantification of HCV infection inc. (e) Quantification of WT or G28A mutant Jc1 infection in Huh-7.5 cells transfected with increasing anti-miR-122 LNA. Values (d,e) represent means and s.d. of triplicate infections. Data were analysed using an unpaired Student’st-test, *P<0.05, **P<0.005, ***P<0.0005. Figure 3: G28A mutation renders Jc1 more resistant to miR-122 inhibition than WT. Analysis of HCV (NS5A) infection by fluorescence-activated cell sorting in ( a ) miR-122 decoy-expressing or naive Huh-7.5 cells transfected with WT or G28A mutant Jc1 RNA, ( b ) naive or miR-122-expressing HepG2 cells transfected with WT or G28A mutant Jc1 RNA and ( c ) Huh-7.5 cells expressing increasing amounts of miR-122 decoy infected with WT (top panels) or G28A mutant (bottom panels) Jc1. ( d ) Quantification of HCV infection in c . ( e ) Quantification of WT or G28A mutant Jc1 infection in Huh-7.5 cells transfected with increasing anti-miR-122 LNA. Values ( d , e ) represent means and s.d. of triplicate infections. Data were analysed using an unpaired Student’s t -test, * P <0.05, ** P <0.005, *** P <0.0005. Full size image HCV (G28A) replicates poorly in the absence of miR-122 We next sought to determine the extent to which miR-122 expression influences replication of the Jc1 G28A mutant. Hepatoma-derived HepG2 cells do not support efficient HCV replication due to the fact that they express very low levels of miR-122; however, they do support efficient HCV replication when engineered to overexpress miR-122 (ref. 14 ). We transfected naive or miR-122-expressing HepG2 cells with WT or G28A Jc1 RNA, and followed viral replication by NS5A flow cytometry analysis. Although HepG2 cells expressing miR-122 supported replication of both HCV RNAs, neither efficiently replicated in naive HepG2 cells ( Fig. 3b ) where miR-122 is not active ( Supplementary Fig. 1b ). These results suggested that replication of the G28A mutant virus was still miR-122 dependent, and led us to hypothesize that this virus replicated in cells expressing the miR-122 decoy because it requires fewer bioavailable miR-122 molecules for efficient replication than WT Jc1 HCV. Sensitivity to miR-122 concentration depends on position 28 To quantify the miR-122 requirements of the WT and G28A Jc1 viruses, we generated a series of Huh-7.5 cell populations with a range of miR-122 activity. To gauge miR-122 activity, we used a miR-122 sensor vector. This is a bidirectional lentiviral vector that coordinately expresses two fluorescent reporter genes, GFP and mCherry, as distinct transcripts. The GFP reporter contains four perfectly complementary miR-122 target sites, whereas the mCherry reporter contains no miRNA target sites ( Supplementary Fig. 1a ). Through this design, all transduced cells are mCherry-positive, while the expression of GFP is inversely proportional to miR-122 activity. Huh-7.5 cells transduced with the miR-122 sensor were mCherry positive and GFP negative, indicating that miR-122 activity is high in these cells. Conversely, Huh-7.5 cells transduced with a miR-142 sensor were both mCherry and GFP positive, demonstrating that miR-142 is not active in these cells, which is expected as they do not express this miRNA ( Supplementary Fig. 1b ). miR-122 sensor Huh-7.5 cells (GFP negative and mCherry positive) were transduced with increasing amounts of the miR-122 decoy vector. In these cells, we observed that miR-122 activity was inhibited even at low decoy dose (as expression of GFP was detectably higher) and inhibition increased in a decoy dose-dependent manner ( Supplementary Fig. 1c ). We next infected these cells with WT or G28A Jc1 and monitored NS5A expression by flow cytometry. Both viruses equivalently infected decoy-negative cells and each virus also showed sensitivity to miR-122 inhibition; however, replication of the WT virus was more sensitive than replication of the G28A mutant ( Fig. 3c,d ). We found a 3.1-fold increase in infection of the G28A mutant above WT Jc1 at the lowest decoy dose tested. To confirm this difference in sensitivity, miR-122 sensor cells were transfected with increasing amounts of a LNA inhibitor targeting miR-122 and infected with either WT or G28A Jc1. As with the decoy, we saw an LNA dose-dependent inhibition of miR-122 activity ( Supplementary Fig. 1d ) and a 2.7-fold increase in resistance to miR-122 inhibition by G28A Jc1 when compared with WT Jc1 ( Fig. 3e ). Using the miR-122 decoy in miR-122 sensor-expressing cells allowed us to derive discrete populations of Huh-7.5 cells with a range of miR-122 activity. Conversely, LNA transfection gave us much more heterogeneous populations of miR-122 activity, which is probably based on transfection efficiency differences ( Supplementary Fig. 1c,d ). Thus, the G28A mutant replicated significantly better than WT Jc1 HCV in the setting of reduced miR-122 bioavailability, suggesting that this nucleotide of the HCV genome influences viral sensitivity to miR-122 concentration. Alignment of the 5′-termini of various HCV reference genomes revealed that naturally many have an A at position 28 ( Fig. 4a ). To assess the relative probability of a G or an A at nucleotide position 28, we analysed ~800 HCV sequences from the Los Alamos National Laboratory United States HCV database ( hcv.lanl.gov ) and found that ~80% of the sequenced HCV genomes contain an A at position 28 ( Fig. 4b ). To determine the sensitivity of different HCV isolates to miR-122 inhibition, we tested the replication of chimeric Jc1 genomes with the 5′-UTR (nucleotides 1–340) of genotype (isolate) 1a (H77), 1b (J4), 2b (J8), 3a (S52), 4a (ED43), 5a (SA13) and 6a (HK6a) in miR-122 decoy or miR-142 decoy (control)-expressing Huh-7.5 cells ( Fig. 4c ). In keeping with previous reports [15] , these chimeras replicated with similar efficiency in Huh-7.5 cells and were not affected by the miR-142 control decoy ( Fig. 4d , dark red and blue bars). However, as observed with the Jc1 virus, all chimeras (J8 and HK6a) with a G at nucleotide 28 were highly susceptible to the miR-122 decoy ( Fig. 4d , light red bars). Conversely, chimeras with an A at nucleotide 28 were only partially affected by the decoy-mediated reduction in miR-122 activity ( Fig. 4d , light blue bars). Furthermore, the degree of resistance to miR-122 knockdown varied between these A28 chimeras. For instance, replication of the chimeric S52 strain was significantly more impaired in miR-122 decoyed cells compared with the other A28 chimeras, whereas the ED43 and SA13 chimeras were most resistant to miR-122 knockdown. To confirm these results, we transfected Huh-7.5 cells with an anti-miR-122 LNA or a control LNA, and infected them with the chimeric Jc1 viruses. Similar to what we found during infection in miR-122 decoy-expressing cells, viruses having the A28 genotype were more resistant to miR-122 antagonism than those having the G28 genotype ( Fig. 4e ). These data indicate that nucleotide 28 is a universal determinant of miR-122 usage, and suggest that other non-miR-122 base pairing elements in the 5′-UTR also dictate HCV’s miR-122 requirement. 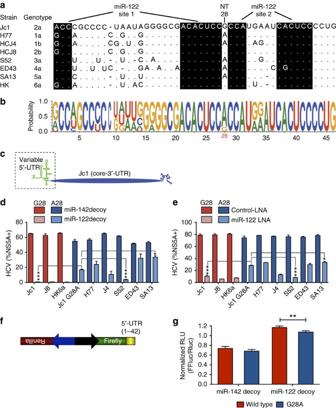Figure 4: Nucleotide 28 in the HCV 5′-UTR is a major determinant of miR-122 usage. (a) Alignment of the 5′-sequences of prototype HCV isolates, Jc1 reference, indicated by strain name and genotype. Black shading indicates miR-122-binding sites and nucleotide 28 of Jc1 is indicated. (b) Relative base probability (represented by letter height) within this region was generated with WebLogo3 using ~800 HCV sequences from the US HCV database (hcv.lanl.gov). (c) Illustration of 5′-UTR chimeras generated. Jc1 5′-UTR chimera infection of Huh-7.5 cells expressing the indicated decoy (d) or transfected with the 1,000 nM of the indicated LNA (e). Strains with G nucleotide 28 are indicated with red bars and strains with A at nucleotide position 28 are indicated with blue bars. (f) Schematic of bidirectional dual luciferase miR-122 reporter bearing the first 42 nucleotides of the HCV 5′-UTR in the Firefly luciferase 3′-UTR. (g) Huh-7.5 cells expressing the indicated decoys were transduced in parallel with equivalent amounts of dual luciferase reporter lentivirus bearing either WT or G28A Jc1 HCV sequence. Shown are ratios of Firefly to Renilla luciferase activity at 3 days post transduction. Values represent means and s.d. of triplicate infections (d,e) and quadruplicate transductions (g). Data were analysed using an unpaired Student’st-test, *P<0.05, **P<0.005, ***P<0.0005. Figure 4: Nucleotide 28 in the HCV 5′-UTR is a major determinant of miR-122 usage. ( a ) Alignment of the 5′-sequences of prototype HCV isolates, Jc1 reference, indicated by strain name and genotype. Black shading indicates miR-122-binding sites and nucleotide 28 of Jc1 is indicated. ( b ) Relative base probability (represented by letter height) within this region was generated with WebLogo3 using ~800 HCV sequences from the US HCV database (hcv.lanl.gov). ( c ) Illustration of 5′-UTR chimeras generated. Jc1 5′-UTR chimera infection of Huh-7.5 cells expressing the indicated decoy ( d ) or transfected with the 1,000 nM of the indicated LNA ( e ). Strains with G nucleotide 28 are indicated with red bars and strains with A at nucleotide position 28 are indicated with blue bars. ( f ) Schematic of bidirectional dual luciferase miR-122 reporter bearing the first 42 nucleotides of the HCV 5′-UTR in the Firefly luciferase 3′-UTR. ( g ) Huh-7.5 cells expressing the indicated decoys were transduced in parallel with equivalent amounts of dual luciferase reporter lentivirus bearing either WT or G28A Jc1 HCV sequence. Shown are ratios of Firefly to Renilla luciferase activity at 3 days post transduction. Values represent means and s.d. of triplicate infections ( d , e ) and quadruplicate transductions ( g ). Data were analysed using an unpaired Student’s t -test, * P <0.05, ** P <0.005, *** P <0.0005. Full size image Adenine at position 28 serves as a better miR-122 substrate To elucidate the mechanism by which nucleotide 28 in the HCV genome has an impact on viral replication in the face of miR-122 inhibition, we sought to characterize how this nucleotide affects miR-122 regulation. To do so, we transduced miR-142 and miR-122 decoy-expressing Huh-7.5 cells with bidirectional dual-luciferase reporter lentiviruses in which the first 42 bases of either the WT or G28A Jc1 5′-UTR were cloned downstream of the Firefly luciferase reporter ( Fig. 4f ). An unregulated Renilla luciferase served as an internal reference. Both WT and G28A Jc1 5′-UTR constructs showed decreased levels of Firefly luciferase in cells expressing the miR-142 decoy (high levels of miR-122 activity) as compared with cells expressing the miR-122 decoy (low levels of miR-122 activity), which confirmed the ability of miR-122 to repress Firefly luciferase linked to the 5′-UTR sequences ( Fig. 4g ). In addition, Firefly luciferase levels were lower in cells transduced with the G28A reporter in comparison with the WT reporter. Although the G28A reporter produced less Firefly luciferase in miR-142 decoy-containing cells than the WT reporter, this difference was only significant in cells where miR-122 activity was limited by decoy expression ( Fig. 4g ). This result parallels the above replication phenotype, where the G28A mutation only enhanced HCV replication in cells in which miR-122 activity is low, and suggests that an A at position 28 may enhance miR-122 accessibility or binding to HCV RNA, which would permit this mutant to replicate efficiently with fewer bioavailable miR-122 molecules. Quantification of miR-122:HCV RNA stoichiometry Our results indicating that HCV replication is highly sensitive to miR-122 bioavailability raised the question of how much miR-122 is needed for HCV replication. The miR-122:HCV stoichiometry in hepatocytes during HCV replication has not been determined. To define this relationship, we first performed quantitative reverse transcriptase–PCR (qRT–PCR) to measure miR-122, HCV and miR-122 decoy RNA copy number in the Huh-7.5 cells expressing increasing levels of miR-122 decoy. In cells expressing no miR-122 decoy, both WT and G28A Jc1 replicated to ~2 × 10 3 HCV RNA molecules per cell, which concurs with previous models and measurements of HCV steady-state replication in Huh-7.5 cells [16] . We found that both WT and G28A Jc1 RNA levels decreased as miR-122 decoy RNA levels increased, but G28A showed a 192-fold increase in HCV RNA levels in comparison with WT at the maximum decoy dose ( Supplementary Fig. 2a ). Although the 192-fold increase in viral RNA in G28A Jc1 was much greater than the 3.1-fold increase that we measured by fluorescence-activated cell sorting, qRT-PCR is more sensitive and quantitative than NS5A staining. In addition, we found that cells expressing increasing quantities of miR-122 decoy had decreased levels of miR-122 ( Supplementary Fig. 2b ), suggesting that the miR-122 decoy not only reduced miR-122 activity but also decreased cellular miR-122 levels, consistent with previous reports from our lab and others [17] , [18] . Combining these data allowed us to show how cellular miR-122 levels relate to HCV replication and enabled us to derive regression equations that approximate the stoichiometry of miR-122:HCV interactions in a cellular context of limiting miR-122 activity ( Fig. 5a ). If we extend this analysis to calculate the number of molecules of miR-122 per cell required to support 1 molecule of HCV RNA per cell, WT HCV required 4,626 molecules of miR-122 per genome, whereas G28A HCV required 3,368 molecules of miR-122 per genome, which is a 1.4-fold decrease ( Fig. 5a , open circles). This calculation was based on conditions of limiting miR-122 activity and was used to assess the relative differences of miR-122 requirements between the WT and G28A viruses. In cells not expressing the miR-122 decoy, we found that WT and G28A HCV require 38.8 and 35.4 copies of miR-122 per genome, respectively (data not shown). 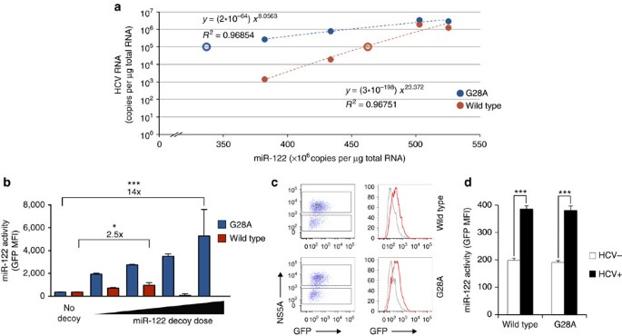Figure 5: G28A Jc1 requires fewer miR-122 molecules for efficient infection than WT. (a) Quantification of HCV and miR-122 RNA in Huh-7.5 cells expressing increasing amounts of miR-122 decoy and infected with G28A (blue dots) or WT (red dots) Jc1. Open dots indicate calculated values for approximation of single-cell miR-122 requirements of G28A or WT Jc1. (b) Quantification of miR-122 activity (GFP mean fluorescence intensity (MFI)) in HCV-positive Huh-7.5 miR-122 sensor decoy cells infected with G28A (blue bars) or WT (red bars) Jc1. As GFP MFI increases, miR-122 activity decreases. Fold change indicates the decrease in miR-122 activity required for total suppression of infection by the indicated virus (14 × for G28 and 2.5 × for WT Jc1). Huh-7.5 miR-122 sensor cells infected with WT and G28A Jc1 show decreased miR-122 activity over uninfected cells, as indicated by increase in GFP (right shift) (c) and GFP MFI (d). Values represent means and s.d. of triplicate infections. Data were analysed using an unpaired Student’st-test, *P<0.05, **P<0.005, ***P<0.0005. Figure 5: G28A Jc1 requires fewer miR-122 molecules for efficient infection than WT. ( a ) Quantification of HCV and miR-122 RNA in Huh-7.5 cells expressing increasing amounts of miR-122 decoy and infected with G28A (blue dots) or WT (red dots) Jc1. Open dots indicate calculated values for approximation of single-cell miR-122 requirements of G28A or WT Jc1. ( b ) Quantification of miR-122 activity (GFP mean fluorescence intensity (MFI)) in HCV-positive Huh-7.5 miR-122 sensor decoy cells infected with G28A (blue bars) or WT (red bars) Jc1. As GFP MFI increases, miR-122 activity decreases. Fold change indicates the decrease in miR-122 activity required for total suppression of infection by the indicated virus (14 × for G28 and 2.5 × for WT Jc1). Huh-7.5 miR-122 sensor cells infected with WT and G28A Jc1 show decreased miR-122 activity over uninfected cells, as indicated by increase in GFP (right shift) ( c ) and GFP MFI ( d ). Values represent means and s.d. of triplicate infections. Data were analysed using an unpaired Student’s t -test, * P <0.05, ** P <0.005, *** P <0.0005. Full size image In previous work, we have shown that the relationship between a miRNA’s concentration and its activity is not always straightforward, as expression differences of some miRNAs do not consistently affect their regulatory abilities [13] . To elucidate how the above differences in miR-122 concentration requirements translate into changes in miRNA function, we sought to determine the activity level of miR-122 required for efficient HCV infection using the miR-122 sensor and decoy cell lines that we established earlier ( Supplementary Fig. 1c ). We infected these cells with WT or G28A Jc1 and quantified NS5A and GFP levels by flow cytometry. We plotted the sensor-based GFP mean fluorescence intensity of infected cells (NS5A positive) in each population to assess the minimal miR-122 activity required for HCV replication. We found that G28A maintains minimal replication capacity when miR-122 is 14-fold less active compared with no decoy conditions, whereas WT HCV replication loses the ability to replicate after a 2.5-fold loss of miR-122 activity ( Fig. 5b ). This 5.6-fold difference in required miR-122 activity between G28A and WT Jc1 indicated that the G28A virus is able to use even less functional miR-122 than the transcript-based stoichiometry would suggest. The fact that we found a difference between these two stoichiometric calculations is not totally surprising given that the decoy reduces miR-122 activity primarily by acting as a sponge, and our transcript-based calculation can only account for the decoy-induced reduction in miR-122 levels. Thus, these data suggest that there is a quantifiable relationship between miR-122 activity and HCV replication, and that viral genetics greatly impact this relationship. HCV infection reduces endogenous miR-122 activity In characterizing the minimal miR-122 activity requirements for efficient HCV replication we found that HCV infection of miR-122 sensor cells, not expressing a miRNA decoy, led to an increase in GFP expression ( Fig. 5c ). We compared the GFP mean fluorescence intensity of the HCV-positive and -negative fractions and found a twofold increase in miR-122-regulated GFP levels ( Fig. 5d ). Although the reduction in miR-122 activity by HCV was less than the inhibition observed with the miR-122 decoy or LNA, it was still surprising considering that our GFP reporter contains four perfectly complementary miR-122 target sites and is a better substrate for miRNA regulation than natural cellular targets of miR-122. These results suggest that the HCV genome sponges miR-122 and reduces its bioavailability. The discovery that miR-122 is an essential host factor for HCV replication altered our view of how this virus interacts with the cell, and represented a new function for a mammalian miRNA [3] . The importance of miR-122 to HCV replication was further highlighted by the impressive response seen in some HCV-infected individuals when treated with anti-miR-122 oligonucleotides [12] . However, many details about the unusual interaction between miR-122 and HCV remain poorly understood, and the variability in patient response to anti-miR-122 inhibitors raised new questions about the relationship between miR-122 and HCV. We showed here that HCV variants actually vary quite significantly in their response to miR-122 inhibition, and that this variation can be attributed, at least in large part, to a single nucleotide change that is found adjacent to but outside of the miR-122 seed-binding sites. These findings provide new insight into HCV’s requirements for miR-122 and have implications for the use of miR-122 inhibitors as a treatment for HCV. Even though all of the patients treated in the Miravirsen trial were infected with genotype 1 HCV, three of the eight individuals at the highest dosage did not exhibit greater than 50-fold reductions in viral loads [12] . Although this difference in response could be due to differences in patient genetics, our data suggest that the genetic diversity in HCV sequence between individuals is likely an important factor. In Lanford et. al. [11] , all of the chimpanzees treated with LNA showed viral rebound after cessation of treatment, and as with the Miravirsen trial no viral escape mutants were reported during or after treatment. Unlike Lanford et. al. [11] who only performed sequencing of the extreme 5′-end of the HCV genome, we sequenced the entire HCV genome and found that no other region of the HCV genome adapts to miR-122 inhibition. This is an important finding because it not only links the effects of anti-miR-122 therapy directly to the 5′-UTR of the HCV genome, but also suggests that mutation in other regions of the HCV genome cannot mitigate anti-miR-122 therapy. In three independent passages of genotype 2a Jc1 HCV through miR-122 decoy cells, we found that the same single nucleotide change (G28A) provided resistance to miR-122 inhibition. Although it is conceivable that we could have passed virus through anti-miR-122 LNA-transfected cells to screen for viruses with resistance to miR-122 inhibition, stable expression of a miRNA decoy within a population of cells provided greater control over miR-122 activity and was probably important for the success of our screen. HCV RNA replication is inherently error- prone, with at least one nucleotide change occurring in every round of synthesis of the RNA genome, which is ~9,000 nucleotides [19] . The G28A variant may have been present in the inoculum, as we used a dose of 1 × 10 5 infectious units; however, the variant may have also arisen during replication after infection. In either case, because the A28 nucleotide confers a replication advantage to the virus under conditions of miR-122 inhibition, the G28A Jc1 was able to outcompete the parent virus. Owing to the high genetic diversity of HCV in a single patient, we would expect this polymorphism to also be present within patients before treatment with any anti-miR-122 therapy. Thus, we would expect the emergence of A28 in individuals infected with HCV strains containing G28. Although we know that miR-122 is highly abundant in bulk liver samples, the expression of miR-122 may vary between hepatocytes and this would give some mutants a replicative advantage. This may account for the higher prevalence of HCV variants with the G28A genotype. Extensive mutation complementation analysis of the interaction between miR-122 and HCV 5′-UTR had not previously identified the importance of nucleotide position 28 (refs 4 , 5 , 6 , 9 ). This is not surprising considering these studies were conducted in cells with high levels of miR-122, and our studies indicate this determinant is only important in cells where the activity of this miRNA is limited. We expanded our study to the other major HCV genotypes, revealing that HCV is sensitive to miR-122 bioavailability in a highly genotype-specific manner, with all genotypes encoding an A at position 28 showing some degree of resistance to miR-122 antagonism. We also found variability in the resistance between genotypes encoding an A at position 28, suggesting that other, yet-to-be-identified bases in the 5′-UTR might affect miR-122 usage. One previous study failed to observe HCV genotype-specific responses to miR-122 inhibition [20] . However, we believe that differences between our experimental setups make a direct comparison of our results difficult. One major difference is that the prior study examined chimeras with the entire HCV 5′-UTR through the non-structural protein 2 swapped between genotypes. Conversely, our chimeric viruses only differed in their 5′-UTRs, while they maintained identical structural and non-structural proteins, which we believe simplifies the comparison between genotypes. In addition, we believe that our positive results stem from the more precise control we exerted over miR-122 activity with our state-of-the-art sensor and decoy lentiviruses. Furthermore, the prior study only assayed the quantity of virus released from treated cells. Our assays examined HCV spread within populations where miR-122 is stably inhibited and, thus, are likely to provide a more sensitive readout of miR-122 dependency. Our analysis indicated that an A at nucleotide 28 did not completely remove HCV’s dependence on miR-122, but did allow the virus to replicate when miR-122 bioavailability was reduced, either due to miR-122 decoy expression or transfection of a miR-122-specific LNA. When we decoupled the WT and mutant miR-122-binding sites from the virus, and placed them downstream of luciferase to study their effect on target regulation, we observed that the reporter linked to the mutant sequence was more suppressed when miR-122 was inhibited. Although this effect was modest, it was impressive considering the sequences only differed by a single non-seed-site nucleotide [21] . Our results suggest that the A at position 28 allows HCV to better scavenge limited quantities of miR-122, most likely by enabling more efficient usage of miR-122. An unanswered question about the miR-122:HCV relationship is just how much miR-122 is required by HCV to replicate. This is important to understand in the development of miR-122 inhibitors, as it could have direct implications on determining the minimal effective dose. Moreover, it has recently emerged that cellular transcripts compete for miRNA ocupancy, and thus that miRNA concentration can be rate-limiting in some contexts [22] . Although miR-122 is highly abundant, it is unknown how much bioavailable miR-122 within hepatocytes is free to interact with HCV. Previous in vitro studies have shown that efficient HCV RNA replication requires binding of two miR-122 molecules to the HCV 5′-UTR [4] , [5] , [6] , [9] . However, these studies do not take into account the other natural cellular targets for miR-122. Our studies indicate that WT Jc1 HCV requires a surplus of cellular miR-122 at a ratio of 1: 38.8. However, when miR-122 decoy is present in cells this ratio jumps to 1:4,626 miR-122 molecules per HCV genome. These calculations relied solely on the total number of miR-122 molecules assessed by qRT–PCR and do not indicate the number of available miR-122 molecules in a cell containing other target sites, especially miR-122 decoy transcripts that primarily act to sequester miRNAs. Thus, the actual ratio of available miR-122 molecules to HCV molecules in a cell may be considerably less. As qRT–PCR-based measurements only account for miR-122 transcript levels, we used a miR-122 sensor to assess miR-122 activity. Using this functional assay, we found that G28A Jc1 required ~5.6-fold less miR-122 activity then WT Jc1, which is four times our qRT–PCR-based calculation. Although each of these calculations has its own inherent caveats and biases, they both agree that G28A requires less miR-122 for replication than WT. Furthermore, the significant genotype-dependent differences in HCV resistance to the miR-122 decoy suggest that differences in the HCV 5′-UTR sequences between genotypes may have an even larger impact on the quantity of bioavailable miR-122 that each virus requires. Interestingly, even in the cells we derived with the highest amount of miR-122 decoy, which contain 30 miR-122 decoy sites for every molecule of miR-122, G28A Jc1 continued to exhibit some capacity to replicate. This is surprising given that the decoy was in overwhelming excess and would be expected to have completely saturated miR-122. Although HCV must compete with cellular targets for miR-122 during infection, we show here that it outcompetes specialized targets such as decoys. This may be explained by the fact that HCV has been shown to actively recruit components of the RNA-induced silencing complex during its replication [23] , [24] , [25] , [26] , and may be a mechanism employed by HCV to recruit miR-122 away from its natural cellular target transcripts. Indeed, we not only found that miR-122 activity affects HCV replication, as expected, but also that HCV infection reduces miR-122 activity—a characteristic suggestive of miRNA sponging by the virus. As miR-122 has been shown to be a potent tumour suppressor gene whose knockout leads to liver inflammation and hepatocellular carcinoma in mouse models [27] , [28] , it is possible that the reduction in miR-122 activity caused by HCV infection could contribute to HCV-associated pathology. Further work will be needed to address this possibility. Taken together, these studies provide quantitative insight into the relationship between miR-122 and HCV, and indicate that the future use of Miravirsen and other miR-122-based drugs for the treatment of HCV infection may need to be tailored according to the HCV sequence being treated. Cell culture 293T, HepG2 and Huh-7.5 (all provided by Charles M. Rice, Rockefeller University [29] ) cells were all grown in DMEM (Gibco) with 100 U ml −1 penicillin, 100 mg ml −1 streptomycin (Mediatech) and 10% fetal bovine serum (Atlanta Biologicals) using standard cell culture techniques [30] . HepG2+miR-122 cells have been described previously [14] . Huh-7.5 cells expressing miRNA decoys have been previously described [13] . HCV and lentivirus generation Lentiviral production was performed as previously described, by cotransfecting three plasmids: (i) a lentiviral provirus encoding the indicated miRNA or miR-decoy, (ii) HIV Gag-Pol and (iii) vesicular stomatitis virus envelope G protein [31] . The HCV Jc1 (ref. 32 ) chimeric virus is genotype 2a and encodes structural proteins and a portion of the NS2 protein from the HC-J6 isolate and the rest of the genome from JFH1 (refs 33 , 34 , 35 ) (provided by Charles M. Rice, Rockefeller University). In short, viral stocks were produced by transfecting Huh-7.5 cells with in vitro -transcribed genomic HCV RNA, collecting supernatants at 2, 3 and 4 days post transfection, and filtering (0.45 μM pore size) before infection assays [30] . HCV infections Huh-7.5 cells were seeded on six-well plates (2 × 10 5 cell per well) 24 h before infection with the indicated virus (multiplicity of infection of 0.1–1). HCV transfection experiments were performed as previously described [14] . For LNA treatment experiments, Huh-7.5 cells containing the miR-122 sensor were seeded on six-well plates (1 × 10 6 cell per well) 24 h before transfection. Cells were transfected with a miR-122 targeting LNA SPC3649 (ref. 11 ): 5′—5TYE665 (fluorophore conjugated to 5′-terminus)—CcAttGTcaCaCtCC (LNA bases are capitalized) (synthesized by Exiqon) using TransIT-X2 (MirusBio) transfection reagent as per the manufacturer’s protocol. Cells were incubated for 24 h at which point the media was changed and incubated for another 24 h. Cells from one well of a six-well plate were then transferred equally into four wells of a 24-well plate and either mock or infected with the indicated virus. Samples were fixed in PBS-4% PFA for 30 min at room temperature 5 days post infection unless otherwise noted, and then stained with anti-NS5A (1:10,000 dilution) (clone 9E10) mouse monoclonal antibody (provide by Timothy Tellinghuisen, Scripps Research Institute and Charles M. Rice) [33] and with goat anti-mouse Alexa-647 (1:500 dilution) (Invitrogen) or Pacific Blue (1:200 dilution) (Invitrogen) secondary antibody. Flow cytometry analysis was performed on the LSR-Fortessa and LSR-II (BD) and analysed using FlowJo. Plasmid construction To generate the G28A mutant Jc1 HCV, PCR was performed to amplify a region of Jc1 between the EcoRI site and the BsiWI site with primers that included this single base mutation. Forward- primer 5′-GACGGCCAGTGAATTCTAATACGACTCACTATAGACCTGCCCCTAATAGGGGCGACACTCCACCATGAATC-3′ and reverse primer 5′-ACACGCATCGCGTACGCCAAGATC-3′. This fragment was then cloned into the Jc1 vector at the EcoRI and BsiWI sites using the In-Fusion HD cloning kit (Clontech) as per the manufacturer’s instructions. To generate the 5′-UTR chimeras, DNA fragments spanning an EcoRI site upstream the T7 RNA polymerase promoter through the entire 5′-UTR (nucleotides 1–340) of each of the indicated genotypes were synthesized (GeneArt Strings, Life Technologies) using published sequences: H77 (accession code: JF343780), HCJ4 (accession code: JF343781), HCJ8 (accession code: JF343783), S52 (accession code: JF343781), ED43 (accession code: JF343785), SA13 (accession code: JF343786), HK6a (accession code: JF343787) [15] . A DNA fragment encompassing the HCV core start codon through the BsiWI site in E1 of Jc1 was PCR amplified using forward primer 5′-CCCGGGAGGTCTCGTAGACCGTGC-3′ and the above-mentioned reverse primer. PCR amplification was performed using the HCV core through BsiWI DNA fragment and the genome-specific GeneArt fragment as the template to create EcoRI through BsiWI fragments for each of the different genotypes using forward primer 5′-GACGGCCAGTGAATTCTAATACGAC-3′ and the above-mentioned reverse primer. This fragment was then cloned into the Jc1 vector using In-Fusion HD cloning. Sensor and decoy-expressing lentiviral vectors were described previously [13] . To generate dual luciferase (Firefly and Renilla) reporters, the first 42 bases of the WT and G28A 5′-UTR were designed and synthesized to contain XbaI-compatible and SalI-compatible overhangs, as well as NheI and AgeI restriction sites at the 5′- and 3′-ends, respectively. Sense and antisense oligos were annealed and ligated into a shuttle backbone, which was digested with XbaI and SalI. 5′-UTRs were then digested with NheI and AgeI cloned downstream of Firefly luciferase in our bidirectional promoter lentviral plasmid [36] , which was digested with NheI and AgeI. Oligonucleotide sequences are as follows: WT_Sense: 5′-CTAGAAGCAGCTAGCACCTGCCCCTAATAGGGGCGACACTCCGCCATGAATCACTCCACCGGTACGAG-3′ WT_AntiSense: 5′-TCGACTCGTACCGGTGGAGTGATTCATGGCGGAGTGTCGCCCCTATTAGGGGCAGGTGCTAGCTGCTT-3′ G28A_Sense: 5′-CTAGAAGCAGCTAGCACCTGCCCCTAATAGGGGCGACACTCCACCATGAATCACTCCACCGGTACGAG-3′ G28A_AntiSense: 5′-TCGACTCGTACCGGTGGAGTGATTCATGGTGGAGTGTCGCCCCTATTAGGGGCAGGTGCTAGCTGCTT-3′. Virus sequencing Viral RNA was extracted from cell supernatants using the QIAamp viral RNA mini kit (Qiagen) according to the manufacturer’s protocol. To perform deep sequencing, extracted RNA was fragmented using the NEBNext Magnesium RNA Fragmentation Module (New England Biolabs) according to the manufacturer’s protocol. Fragmented RNA was then prepared for high-throughput sequencing on the Illumina platform using the ‘TruSeq RNA Sample Preparation Kit v2’ (Illumina Inc.) according to the manufacturer’s protocol with the RiboZero and poly-A capture steps being skipped. Samples were sequenced on a HiSeq2000 sequencer (Illumina Inc.). To sequence the 5′-end of the HCV genome, the 5′-rapid amplification of cDNA end system for rapid amplification of cDNA ends kit (Life Technologies) was used following manufacturer’s protocol. The primers used were as follows: GSP1: 5′-TGGTGATGCAGGACAGCAGG-3′, GSP2: 5′-CCGCCCGGAAA CTTAACGTCTTGT-3′, GSP2’: 5′-GTGTTTCTTTTGGTT TTTCTTTGAGGTTTAGGA-3′. Sequences were aligned using BWA-MEM and base counts at each reference position were created using samtools ‘mpilieup’ version 0.1.19 (ref. 37 ). To avoid spurious calls, indels and bases with quality lower than Q13 ( P -value>0.05) were excluded from analysis. RNA quantification for stoichiometry Total RNA was extracted from cells using Qiazol (Qiagen) according to the manufacturer’s instructions. RNA concentration was determined by 260/280 nm optical absorbance using a NanoDrop 2000 spectrophotometer (Thermo Scientific). miRNA analysis was then performed as previously described [18] , using a standard curve generated from a synthetic miR-122 RNA (5′-UGGAGUGUGACAAUGGUGUUUG-3′, Integrated DNA Technologies). HCV RNA quantification and qRT–PCR were performed as previously described [38] . To determine miR-122 decoy mRNA levels, reverse transcription was carried out with 1 μg total RNA using the high-capacity RNA-to-cDNA kit (Applied Biosystems). qPCR analysis of miR-122 decoy was performed using the SYBR green qPCR master mix 2 × (Fermentas, Thermo Scientific) using the following primers: 5′-GACGGCGCTAGGATCATCAAC-3′ and 5′-ATTCTGTGACCAGAATAC-3′. We quantified the absolute concentration of decoy transcripts as previously described [18] . Briefly, we generated a standard curve using in vitro -transcribed decoy mRNA. To do this, we linearized a pBlue plasmid containing the miR-122 decoy upstream of a T3 site, and performed in vitro transcription using the MEGAscript T3 Kit (Ambion). The resulting RNA was purified by RNeasy (Qiagen), visualized on a gel to confirm the correct product size and quantified by NanoDrop. Twofold Serial dilutions of the RNA were made into 1,000 ng of unrelated total RNA starting from 240 pg RNA per μg total RNA to 0.234 pg per μg total RNA. Samples were analysed on an ABI Prism 7900HT Real Time PCR System. Three technical replicates and three biological replicates were carried out for each experiment. Statistical analysis Data were analysed using an unpaired Student’s t -test, * P <0.05, ** P <0.005, *** P <0.0005 on Prism software (GraphPad Software). Values in graphs represent the mean and s.d. of representative experiments performed in triplicate or quadruplicate. How to cite this article: Israelow, B. et al. Hepatitis C virus genetics affects miR-122 requirements and response to miR-122 inhibitors. Nat. Commun. 5:5408 doi: 10.1038/ncomms6408 (2014). Accession codes: The viral RNA sequence data have been deposited in the NCBI Sequence Read Archive (SRA) under accession code SRR1588185 .